Power-independent wavelength determination by hot carrier collection in metal-insulator-metal devices Wavelength separation and detection is generally performed by spatial dispersal of incident light onto separate detectors, or by appropriate wavelength-selective filters. Here we demonstrate direct wavelength determination of monochromatic light in a power-independent fashion with a single metal-insulator-metal device. This simple platform allows facile fabrication and scaling, and may be useful for on-chip optical communications. Although a single wavelength is power-independent, with two or more concurrent input signals, the output obeys a simple current sum rule, allowing the output to be tuned by choosing the input wavelengths and power. Finally, we demonstrate real-time deconvolution of three different wavelength asynchronous signals. Since Newton first demonstrated dispersion of white light into its separate components [1] , photon wavelength is typically determined by dispersing the light then measuring the intensity as a function of location, or by use of wavelength-selective resonators or filters. Wavelength determination and selection is crucial in many applications, such as wavelength division demultiplexing for optical communication systems, sensing systems, tunable diode lasers and even for emerging optical interconnects and plasmonic nanocircuits [2] , [3] , [4] , [5] , [6] , [7] . For communications applications, it is not only critical to separate the individual wavelength signals but also to monitor their temporal signal intensity. Several recent studies have investigated alternative methods for wavelength measurement, including quantum well photodetectors [8] , macrobending single-mode fibres [9] and metal-semiconductor-metal photodetectors [10] . However, these devices require at least two differently tuned detectors, with one acting as a reference to remove power-dependent effects. Each individual photodetector gives rise to a photocurrent signal that varies with incident power, making it unsuitable for wavelength detection by itself. Here we show that the quantum mechanical information about the incident photon energy is stored within ballistic hot electrons upon absorption, which can be read-out by a simple metal-insulator-metal (MIM) junction. Photo-absorption within the upper metal electrode creates hot carriers with energies up to the incident photon energy, which may emit into the conduction band of the insulator through internal photoemission (IPE; Fig. 1 ). In this device, the open-circuit voltage ( V oc ) between the upper and lower electrodes is directly proportional to the energy difference between the hot electron and the metal-insulator band offset and is not dependent on incident power. To our knowledge, this is the first report that the V oc can be reliably used as a power-independent wavelength detector. In general, photoexcited hot carrier extraction has recently proven to be a fertile area for solar energy collection [11] , [12] and photodetection [13] , [14] , and can take advantage of plasmonic absorption enhancement in metal films [15] . IPE processes are also used within semiconductor homojunctions as a mechanism to lower the minimum cutoff energy for far-infrared detectors [16] , [17] . 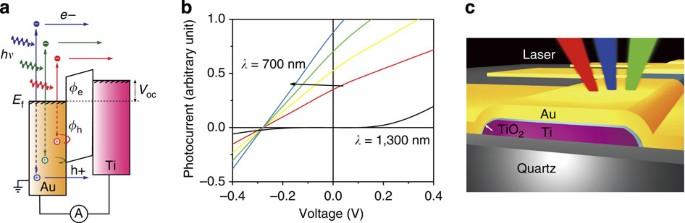Figure 1: Schematic of the MIM device with its energy diagram. (a) Energy diagram of Au–TiO2–Ti device. Photons excite electrons to higher energy levels, which provide them with enough energy to traverse the barrier. Hot electrons and holes are represented by solid and hollow circles, respectively. (b) Calculation of photocurrent with barrier heightsφeandφhbeing 1.0 and 2.0 eV, respectively. Power change from 1.0 to 2.5 mW with 0.5 mW difference along the arrow has no influence on the open-circuit voltage at 700 nm. No open-circuit voltage at 1,300 nm. (c) Schematic of three lasers illuminating MIM devices on quartz substrate simultaneously. Figure 1: Schematic of the MIM device with its energy diagram. ( a ) Energy diagram of Au–TiO 2 –Ti device. Photons excite electrons to higher energy levels, which provide them with enough energy to traverse the barrier. Hot electrons and holes are represented by solid and hollow circles, respectively. ( b ) Calculation of photocurrent with barrier heights φ e and φ h being 1.0 and 2.0 eV, respectively. Power change from 1.0 to 2.5 mW with 0.5 mW difference along the arrow has no influence on the open-circuit voltage at 700 nm. No open-circuit voltage at 1,300 nm. ( c ) Schematic of three lasers illuminating MIM devices on quartz substrate simultaneously. Full size image Device principles Unlike photocurrent, which is highly dependent on the illumination power, the open-circuit voltage in a MIM hot electron device depends upon the energy of the incident photon. The process is based on the physics of IPE, which has been extensively reviewed. Briefly, when an MIM device is illuminated from above, more photons are absorbed in the upper electrode than in the lower electrode ( Fig. 1a ). This creates a population of ‘hot’ carriers with a maximum excitation equal to the photon energy. Assuming that carriers propagate isotropically in all directions, half of the excited carriers will travel towards the metal-insulator interface. For materials such as Au and Ag, the electron mean free path can be on the order of 50 nm [18] , so that for thin metal electrodes an appreciable fraction of photoexcited electrons can reach the surface before scattering. When they reach the interface, as shown in Fig. 1a , hot electrons that have energies greater than the electron barrier φ e will cross the barrier through the conduction band of the insulator, generating a positive forward photocurrent, whereas hot holes can generate reverse photocurrent. Similarly, hot electrons generated by absorption within the lower electrode will travel from the bottom to the top electrode, reducing the forward current. Hot electrons with lower energy than the interface barrier either recombine or reflect at the interface and lose energy through collisions, and are assumed not to contribute to the current. The open-circuit voltage ( V oc ) occurs at the zero photocurrent point (after removing dark current), which is achieved by applying negative bias to increase the electron barrier height of the opposite electrode. When the total barrier energy equals the incident photon energy, the current should drop to zero for monochromatic illumination, ignoring the effects of hot holes and reverse current (which can be significant depending on the device geometry). This voltage is dependent upon the photon energy, but not illumination power. The theoretical I – V response for two different wavelengths of light, 700 and 1,300 nm, in an MIM device with an electron and hole barriers, φ e and φ h of 1.0 and 2.0 eV, respectively, is shown in Fig. 1b . For low-energy photons, no electrons are excited over the barrier (1,300 nm, 0.95 eV), and the IV curve is flat. For photons with energy greater than the barrier height (700 nm, 1.77 eV), the short-circuit photocurrent ( V =0) increases with intensity, however the V oc ( I =0) remains fixed. The V oc can be calculated from the incident photon energy, the electron barrier energy and the ratio of photocurrent generated in the top versus bottom electrodes [11] : where I sc and V oc are short-circuit current and open-circuit voltage, respectively. Note that if , then , as is the case for strong optical absorption in the upper electrode [15] . As shown in Fig. 1b , increasing the illumination power change does not affect the open-circuit voltage. The device materials should be carefully selected to have proper band alignments at the metal-insulator interfaces ( Supplementary Fig. S1 ). To test these concepts in operation, we fabricated thin film Au–TiO 2 –Ti junctions as diagrammed in Fig. 1c . A 30-nm thick electron-beam-evaporated Ti film was deposited as the bottom electrode, followed by oxygen plasma oxidation to form a high-quality TiO 2 -insulating layer. A 40-nm thick Au layer was then deposited as the top layer, chosen for the relatively low (0.9 eV) Au–TiO 2 interfacial conduction band offset, ensuring a long wavelength detection cutoff [19] . Because of the band offset, TiO 2 acted as an insulator within the junctions, with the typical oxide thickness of 7.4 nm [20] ( Supplementary Fig. S2 ) based on a Simmons model fit to the I – V curve. Typical junction areas were 90 × 130 μm 2 . Power-independent open-circuit voltage The MIM performance was assessed from the current-voltage responses for different illumination intensities over a wavelength range of 450–1,600 nm. 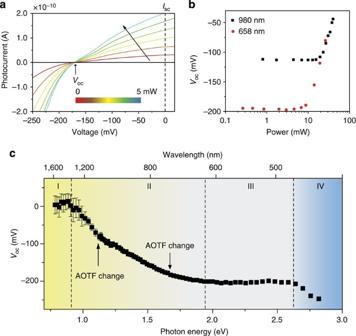Figure 2: Wavelength determination by unique power-independent open-circuit voltage. (a) Photocurrent under bias illuminated with 808 nm laser at different power showing constant open-circuit voltages. (b) Response ofVocat different wavelengths showing wide range of power independence. (c)Vocin the wavelength range from 450 to 1,600 nm. Region I: 1310–1600, nm,Vocis zero as the photon energy is lower than the barrier height. Region II: 650–1310, nm, linear wavelength determination region. Region III: 490–650 nm, almost constantVocdue to hole injection. Region IV: 450–490 nm, increasing and power-independentVocdue to absorption in TiO2. Figure 2a shows the I–V traces for monochromatic illumination at 808 nm. The current is positive at voltages greater than the V oc , with a roughly linear response within quadrant II. As the power increases from 0.73 to 4.51 mW, the I–V slope increases dramatically, with short-circuit currents (the current at zero potential) rising proportionately from 0.23 to 1.3 μA cm −2 . However, the open-circuit potential ( V oc ) of −170.5±0.5 mV changes less than the noise (0.5 mV) for all intensities, demonstrating the power-independent nature of the V oc in these devices. Although the slope of a linear IV is typically equated to an ohmic resistance, the physical identify of the resistive element is more subtle in this case. As decreasing current arises from electron reflection back into the metal followed by energy loss, the power dissipation occurs within the metal, not the insulating layer. Overall, the response reflects the overall junction resistance of the MIM device, and not a particular layer. Figure 2: Wavelength determination by unique power-independent open-circuit voltage. ( a ) Photocurrent under bias illuminated with 808 nm laser at different power showing constant open-circuit voltages. ( b ) Response of V oc at different wavelengths showing wide range of power independence. ( c ) V oc in the wavelength range from 450 to 1,600 nm. Region I: 1310–1600, nm, V oc is zero as the photon energy is lower than the barrier height. Region II: 650–1310, nm, linear wavelength determination region. Region III: 490–650 nm, almost constant V oc due to hole injection. Region IV: 450–490 nm, increasing and power-independent V oc due to absorption in TiO 2 . Full size image The V oc as a function of incident power for two wavelengths, 658 and 980 nm, is shown in Fig. 2b . The V oc for both wavelengths remains constant over nearly two orders of magnitude at values of −195.8±0.9 and −112.7±0.5 mV, respectively, until two-photon processes become important around 10 mW ( Supplementary Fig. S3 ). Power-independent V oc ’s were observed for all wavelengths >460 nm ( Supplementary Fig. S4 ), at which point a distinct V oc decrease is observed with increasing power, as described below. The variation of V oc with power is <2% for the worst-case photon energy, and more often <0.5%. The value of the V oc as a function of photon energy is shown in Fig. 2c , demonstrating that the photon wavelength can be uniquely determined solely based on an electrical measurement. However, there is a limit to the useful V oc -wavelength response regime based on the band offsets within the MIM junction. The broadband V oc response from 450 to 1,600 nm has four distinct regions, labelled as I, II, III and IV, in Fig. 2c . In region I from 1,310 to 1,600 nm, V oc is zero and flat as a function of photon energy. In this regime, the photon energy is lower than the Au–TiO 2 band offset, and only a small amount of electron tunnelling contributes to the current, insufficient to create a measureable V oc . The transition to region II at 0.95 eV (1310, nm) is in good agreement with the Au–TiO 2 interface barrier height measured from the device I – V curves, 0.87 eV ( Supplementary Fig. S2 ), as well as that reported by McFarland et al . (0.9 eV) [19] and Marri et al . (0.87 eV) [21] . In the wavelength-sensing region II from 650 to 1,310 nm, V oc varies monotonically with photon energy as a larger voltage is required to prevent the more energetic hot carriers from injecting into the TiO 2 . Each voltage corresponds to a unique wavelength, allowing wavelength determination throughout this region. Note that the slight discontinuities of the V oc curve at 750 and 1,100 nm is caused by switching of acousto-optic tunable filters (AOTF) crystals within the laser. In region III, the photon energy becomes greater than the hole barrier, φ h . In this case, the hot holes in the top metal contribute to a backward photocurrent that negates further additional forward current as photon energy increases [11] . As the photon energy increases above φ h , equal numbers of additional electrons and holes are generated with sufficient energy to cross the MIM insulator barrier [22] . These equal positive and negative current contributions cancel, and as a result the additional photo-generated hot carriers excited by photons with energy larger than φ h make no contribution to the open-circuit voltage. The V oc versus wavelength in this region is therefore flat, with a nearly constant at a value of −198±2 mV. Note that there is a slight decrease in the absolute value of the photovoltage at around 500 nm, which we attribute to increased light penetration into the lower Ti electrode, leading to larger backward photocurrent [15] . The transition from region II to region III occurs at ~650 nm, corresponding to a hole barrier energy height φ h of 1.9 eV. The bandgap of the TiO 2 thin film is the sum of φ e + φ h =2.85 eV, which is smaller than bulk anatase crystalline TiO 2 , but consistent with TiO 2 formed by Ti oxidation, where oxygen vacancies have led to band gaps of 2.55 and 2.81 eV [23] , [24] . In region IV, the V oc decreases as the photon energy reaches the bandgap of the TiO 2 . At these wavelengths, the broad absorption edge of TiO 2 causes photoexcitation within the insulator itself, directly contributing to the forward photocurrent and decreasing the V oc . As the wavelength decreases, the optical absorbance becomes stronger, changing the V oc more rapidly as observed at 460 nm ( Supplementary Fig. S4 ). The largest detection wavelength ranges are thus achieved by using an insulator with a large bandgap and large hole barrier (valence band offset). The wavelength resolution of the MIM device depends on the precision of the open-circuit voltage determination. At long wavelengths (for example, in the near-infrared region) where photon absorption in Au is very low and the photon energy is close to the barrier height (resulting in fewer carriers with sufficient energy to cross the MIM barrier as the percentage of hot electrons that can inject into the conduction band of insulator is approximately to be φ e / E ph , where E ph is the photon energy, as the energy distribution of hot electrons above Fermi level is approximately uniform), the V oc determination was limited because of noise. We define the wavelength resolution to be the V oc uncertainty divided by the average slope in region II (0.28 mV nm −1 ). In the case of 808 nm diode laser illumination, the resolution is as fine as 1.8 nm due to the high illumination power. At a much lower power and longer wavelength (for example, 0.15 mW at 1,020 nm using a Fianium supercontinuum laser), the noisier photocurrent leads to larger V oc uncertainty, giving rise to a V oc =−108.8±5 mV and a resolution of ±17.8 nm. However, by increasing the photon absorption in the upper electrode, such as through surface plasmon enhancements that can increase absorption by over an order of magnitude, the resolution could be improved to better than ±1 nm. Open-circuit voltage under two-laser illumination Although most IPE treatments consider a single wavelength, an interesting situation arises when two or more different wavelengths simultaneously illuminate the sample. Excluding the two-photon processes that occur at higher power, each wavelength above the electron barrier height should contribute to the total current in a voltage-dependent fashion. Assuming that the photocurrent-voltage response in region II for a given wavelength can be modelled as a linear function ( Supplementary Fig. S5 ), the current from V oc to 0 bias can be expressed as: Where m i is respective photocurrent slope (photo-conductance) in the range of [ V i , 0] under the i th illumination wavelength, I sc is the short-circuit current, and V i is the corresponding open-circuit voltage. Note that the slope m i for each wavelength will be power dependent, as shown in Fig. 2a . The total current is found from a simple current sum rule, which is solved to find the combined V oc : We investigated the validity of this simple analysis by testing the MIM photocurrent response for two simultaneous illumination of 808 and 980 nm ( Fig. 3 ). Photocurrent-voltage curves were measured by holding the power at 980 nm constant, and systematically increasing the intensity at 808 nm. As the power at 808 nm increases, the open-circuit voltage varies with the new nodal point changing between −160.6 and −121.6 mV as shown in Fig. 3a , blue squares. The expected V oc for dual wavelength illumination is plotted in Fig. 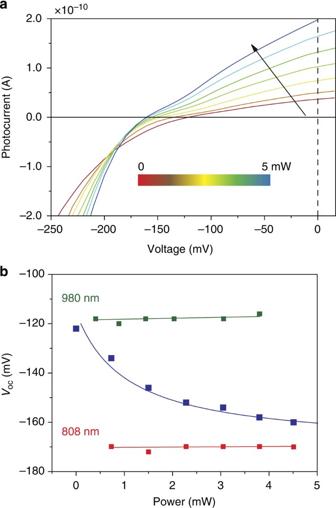Figure 3: Power-tunedVocunder dual wavelength illumination. (a) Photocurrent as a function of bias under illumination at 808 and 980 nm. The power at 808 nm is modulated while the power at 980 nm is kept constant. (b)Vocunder dual wavelength laser illumination compared with single laser illumination. A model (blue curve) based on photocurrent data is in excellent agreement with the experimental results (blue squares). 3b (blue curve) according to: Figure 3: Power-tuned V oc under dual wavelength illumination. ( a ) Photocurrent as a function of bias under illumination at 808 and 980 nm. The power at 808 nm is modulated while the power at 980 nm is kept constant. ( b ) V oc under dual wavelength laser illumination compared with single laser illumination. A model (blue curve) based on photocurrent data is in excellent agreement with the experimental results (blue squares). Full size image where m 1 and m 2 are the respective photocurrent slopes, and V 1 and V 2 are the V oc values at 808 and 980 nm, respectively. m 1 is linearly dependent on the power ( Supplementary Fig. S6 ). The theory is in excellent agreement with the experimental results, even though the calculated V oc was predicted solely on the individual 808 and 980 nm photocurrent data, and not a fitted curve. Thus, even for multispectral signals it is possible to accurately predict the total V oc if the response for each individual wavelength is known. Once the V oc and slope values were determined, no additional knowledge of the input signals was necessary. However, given the number of variables, this technique is likely not appropriate for detection of broadband illumination of arbitrary intensity. Asynchronous signal deconvolution As an example of the multispectral response, we examined real-time deconvolution of simultaneous multi-wavelength signals at a single location without spatial separation or filtering of the signals. Such a situation may occur within communication-type applications, where a finite number of light sources with known characteristics are incident at a single location. As shown in schematically in Fig. 1c , a MIM device was illuminated simultaneously by three lasers with wavelengths at 600, 808 and 980 nm ( Supplementary Fig. S7 ). The IV curve for each wavelength was initially measured independently ( Fig. 4a ) to derive the V oc and slope for each wavelength. These three wavelengths were then chopped at different rates, altering the combination of signals at any given time, and simultaneously illuminated onto the sample. The open-circuit voltage is then detected in real-time using a Keithley sourcemeter ( Fig. 4b ). 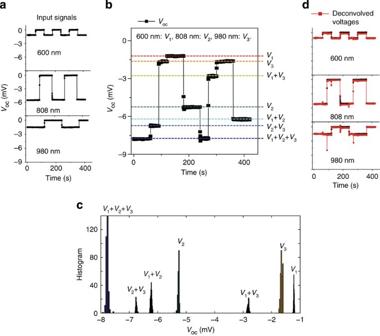Figure 4: Deconvolution of multiple signals. (a) Input asynchronous laser signals at individual wavelengths. (b) Output signal of a single MIM device illuminated by three lasers chopped at different rates. (c) Histograms of measured voltages under different illumination combination. (d) Deconvolved results (red squares) are in excellent agreement with the input signals (black squares) at 600, 808 and 980 nm. Figure 4: Deconvolution of multiple signals. ( a ) Input asynchronous laser signals at individual wavelengths. ( b ) Output signal of a single MIM device illuminated by three lasers chopped at different rates. ( c ) Histograms of measured voltages under different illumination combination. ( d ) Deconvolved results (red squares) are in excellent agreement with the input signals (black squares) at 600, 808 and 980 nm. Full size image From the characteristic open-circuit voltage at different times, the original separate input signals could be deconvolved. With the three asynchronous signals, the output signal varied with time as shown in Fig. 4b . Each distinct voltage level corresponds to different combinations of the three input signals. For example, during the first 60 s, all three signals are on with a maximum output voltage of −7.75±0.018 mV, which indicates the combination of all three signals. There are seven clearly defined voltage levels in total, as noted by the V 1 , V 2 and V 3 notation for each wavelength. In Fig. 4c , the histogram of each level shows a narrow voltage distribution, indicating the good uniformity and selectivity. From the standard deviations of each signal, the probability that a particular measurement was actually a result of another combination of signals was extremely low. For the closest signal levels, V 1 and V 3 , the probability of incorrectly identifying the proper signal was lower than 10 −10 based on a Student’s t- test analysis, which indicates a clear distinctness between V 1 and V 3 . The asynchronous signal in each wavelength channel was then deconvolved from the measured voltage levels, as shown in Fig. 4d , red squares. Figure 4d is a plot of the input signals together with the deconvolved results that show excellent agreement. The confidence levels are all >99.99% at all wavelengths, such that each signal comes from an independent source, demonstrating the high accuracy of the deconvolved results compared with the input signals. In summary, we have demonstrated monochromatic wavelength determination and polychromatic deconvolution at a single site with a single, easily fabricated MIM device. Different wavelengths of light, with energies in the range from φ e to φ h , are each detected according to their power-independent open-circuit voltages. Using this MIM device, multiple signals can be demultiplexed at a single location. There are two other intriguing aspects to these devices that have not yet been explored. One is that because the ballistic electron transport process is extremely fast (~order ps), the devices could operate at high frequencies. The relaxation of hot electrons in the metals similarly occurs in ps, eliminating residual current after a light pulse. The second is that unlike photocurrent, the V oc is independent of device area; thus in principle these could be scaled to nanometre dimensions without affecting the measurement. In practice, we are currently limited by amount of current necessary to measure the V oc , yet with improved light-coupling techniques, this could be significantly improved. For example, periodic grooves or scattering centres on the Au electrode to couple light into surface plasmons should greatly strengthen the signal, resulting even better sensitivity and wavelength resolution. Future development of electrode and insulating materials with small electron barriers and a large hole barriers (allowing electron injection but blocking holes) will also expand the wavelength-determination range. Because of their small size and ability to handle many signals at once, these devices may be applied to future optical communications and on-chip optical interconnects. Calculation of photocurrent To calculate the photocurrent-voltage characteristics, we first obtained the probability of photoexcitation at the different positions within the MIM devices. The excitation probability is dependent on metal dielectric constants and the volumetric absorbance η ( z ), which is defined to be , where S ( z ) is the photon flux in the devices as a function of position, S 0 is the incident flux. The flux in the devices was obtained based on two-dimensional simulation finite-difference frequency-domain methods. After photoexcitation, half of the hot electrons were assumed to move towards the metal-insulator interface, whereas the other half moved towards the top surface and are assumed to decay. The probability that hot electrons moving towards the junction reach the metal-insulator interface follows exp(− δz/λ ) where δz is the distance from the interface, and λ is the mean free path of hot electrons in the metal [25] . As the hot electrons reach the metal-insulator interface, the transmission probability through the barrier was assumed to be unity for electrons with energies larger than the barrier height. Electrons with energy below the barrier have tunnelling probability calculated by WKB approximation [26] . The barrier shape varies linearly with the applied voltage, which changes the transmission probability correspondingly. The total photocurrent is the sum of the positive forward photocurrent from top metal to the bottom metal and the negative backward photocurrent from bottom metal to the top metal. Sample preparation Au–TiO 2 –Ti devices were fabricated on fused quartz substrates. The substrates were cleaned in Piranha solution and rinsed with de-ionized water. Thirty-nanometre thick titanium bottom electrodes were deposited on the substrates using electron beam evaporation with a shadow mask. These electrodes were treated with O 2 /Ar (10:90) plasma etching for 15 min to form a thin layer of TiO 2 . A layer of Au with a thickness of 40 nm was deposited on top of Ti/TiO 2 by the evaporation through a shadow mask to form the cross-junction. Finally, the devices were wire-bonded to a chip carrier for the electrical and optical measurement. Experimental setup Photocurrent was recorded by a SR810 lock-in amplifier together with a SR570 low-noise current preamplifier. The voltage was controlled by a Keithley 2612 sourcemeter, while Fianium supercontinumm laser provided illumination from 450 to 1600, nm. The laser power was measured by a NOVA II power meter. The laser was focused with a × 50 objective, and the position of the laser spot on the devices was monitored by a CCD (charge-coupled device) camera. Another two diode lasers at wavelengths of 808 and 980 nm were used for the multi-illumination measurement. During the signal deconvolution, the 600 nm light was from the Fianium laser. The three lasers were chopped at different rates mechanically before shining on the devices and all of them were focused by the same objective. For signal deconvolution, the voltages are measured directly by the SourceMeter without the lock-in amplifier. The voltage measured in this way is the value when the photocurrent is equal to the dark current. As a result, the voltage directly measured by the SourceMeter for two-light illumination does not follow equation (1) but obeys an approximate voltage sum rule. These measured voltages are smaller than the characteristic V oc at each wavelength and are power dependent under multi-illumination. However, as long as the input power is known, each voltage still corresponds to one wavelength and can be converted to its characteristic photovoltage. How to cite this article: Wang, F. & Nicholas, N. A. Power-independent wavelength determination by hot carrier collection in metal-insulator-metal devices. Nat. Commun. 4:1711 doi:10.1038/ncomms2728 (2013).